Epithelial organisation revealed by a network of cellular contacts The emergence of differences in the arrangement of cells is the first step towards the establishment of many organs. Understanding this process is limited by the lack of systematic characterization of epithelial organisation. Here we apply network theory at the scale of individual cells to uncover patterns in cell-to-cell contacts that govern epithelial organisation. We provide an objective characterisation of epithelia using network representation, where cells are nodes and cell contacts are links. The features of individual cells, together with attributes of the cellular network, produce a defining signature that distinguishes epithelia from different organs, species, developmental stages and genetic conditions. The approach permits characterization, quantification and classification of normal and perturbed epithelia, and establishes a framework for understanding molecular mechanisms that underpin the architecture of complex tissues. Investigating the interactions between components as a network provides a common platform to uncover signatures of complex systems [1] , [2] , [3] , [4] , [5] . While this approach has been recently exploited to investigate biological systems of different scales, ranging from interactions between molecules to interactions between species, application of network theory at the level of individual cells has been rather limited. In this study, we present a network-based approach to understand general principles in the organisation of cells in an organism (that is, epithelia). Early in animal development, cells in an epithelia begin to divide and alter their position, shape and size in stereotypical ways [6] , [7] , [8] , [9] , [10] , [11] , [12] , [13] , [14] , [15] . Despite being a highly dynamic process, this results in ordered, robust structure that ultimately leads to the formation of mature organs with cellular organisation suited to their specialised functions. Though we have an understanding of the contribution of genetic mechanisms (for example, external signals and the associated gene regulatory pathways [6] , [14] ) and cellular mechanics (for example, intrinsic patterns arising due to the rate of cell division [8] , [9] , [11] , [15] or cell rearrangement due to anisotropy of cortical forces within individual cells [6] , [16] , [17] , [18] , [19] , [20] ) to the development of epithelial architecture in various model systems, we lack the means to objectively characterise and quantify the similarities and differences in the organisation of epithelia. Previous studies have offered insights into epithelial organisation by focusing primarily on geometric characteristics of individual cells such as the cell area and the number of contacts [8] , [9] , [18] , [21] , and have led to the formulation of empirical relationships such as Aboav-Weaire's law and Lewis's law [22] , [23] . This has largely emphasised the similarity between different epithelia. However, a more comprehensive view of epithelial organisation can be achieved if one considers the higher order organisation of cells such as the patterns in the network of interactions between cells that typically characterises an epithelium. The ability to do this would provide a way to describe objectively an epithelium, facilitate the investigation of fundamental questions about its organisation and dynamics, and establish an objective basis for comparative studies of epithelia from different sources. Importantly, the network characteristics of epithelial organisation (as opposed to geometric features) are not readily assessed by eye. This implies that higher-order organisation may not be accounted for in our current understanding of epithelial architecture. In this work, we present an approach we term GNEO (geometric and network representation of epithelial organisation), which by combining network and geometric measures of epithelial organisation addresses these issues. We show that our approach is able to capture a defining signature that distinguishes epithelia from different organs, species, developmental stages and genetic conditions. In this way, GNEO permits characterisation, quantification and classification of normal and perturbed epithelia in an objective manner. The GNEO method for characterising epithelial organisation In order to capture information about the spatial organisation of cells and the global features of an epithelium, we generated network representations of confocal images of epithelia based on cell–cell contacts. This allows principles from graph theory and complex networks [2] , [3] , [5] , [24] to be used to investigate short- and long-range patterns in epithelial organisation. In such a network, the centre of each cell is treated as a node and two nodes are linked if the two cells are neighbours (that is, physically contact each other) in the epithelium (Methods; Fig. 1a ; Supplementary Fig. S1 ). For each image, we generated a 'feature vector' consisting of eight features ( Box 1 ): the means and s.d. 's of the cell area, degree (that is, number of neighbours), clustering coefficient (the amount of interconnectedness among a cell's immediate neighbours) and average degree of neighbours (the average number of neighbours of a cell's neighbour). Thus, the mean values of the features in the feature vector represent information about the cell shape (area and degree) and the pattern of cell-to-cell contacts (degree, clustering coefficient and average degree of neighbours). While the degree is informative of the short-range pattern of contacts (the immediate neighbours of cell), the clustering coefficient and average degree of the neighbours represent the cell's context and surrounding, thus reflecting higher-order organisation. In turn, the s.d. values are indicative of the cell-to-cell variability (that is, heterogeneity) of a feature in an epithelium. 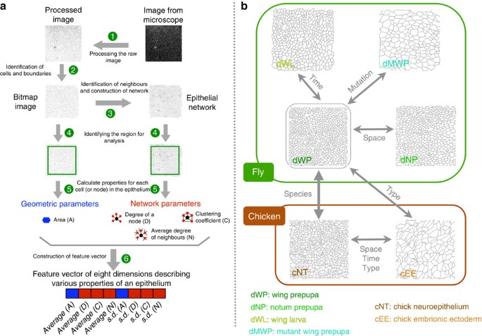Figure 1: GNEO approach and epithelial comparisons performed. (a) GNEO approach to characterise epithelial organisation. (1) Images from the confocal microscope are processed to get a light background with dark cell contours. (2) The processed image is the source for defining individual cells, as well as for determining the number of neighbours for every cell. (3) This information is used to produce an epithelial network where each cell is represented as a node, and the two nodes are connected if the two cells are neighbours in the epithelium. (4) A region of interest (ROI; shown in a green box) is selected for further analysis and the cells that border the ROI are excluded. (5) The average and s.d. of area and three network features over all cells in an epithelium are calculated. (6) This information is represented as a feature vector, which is an eight-dimensional vector that characterises each epithelium. Each of the four features considered in this work is abbreviated by the symbols shown in this figure. (b) Schematic representation of the comparisons of epithelia from different sources performed in this study. Images of representative epithelial samples (2-pixel wide cell contour) fromDrosophila(different tones of green labels, fly) and chick (different tones of brown labels) are shown. The reference prepupal wing pouch epithelium is shown within a grey box. The text in grey denotes the relationship between epithelia from the different sources that were compared.Space: spatially separated epithelia from the same organism;time: temporally separated epithelia from different stages of development;type: different types of epithelia (that is, squamous and columnar);species: epithelia from different organisms (vertebrate (chick) and invertebrate (Drosophila)) andmutation: mutant epithelia. Figure 1: GNEO approach and epithelial comparisons performed. ( a ) GNEO approach to characterise epithelial organisation. (1) Images from the confocal microscope are processed to get a light background with dark cell contours. (2) The processed image is the source for defining individual cells, as well as for determining the number of neighbours for every cell. (3) This information is used to produce an epithelial network where each cell is represented as a node, and the two nodes are connected if the two cells are neighbours in the epithelium. (4) A region of interest (ROI; shown in a green box) is selected for further analysis and the cells that border the ROI are excluded. (5) The average and s.d. of area and three network features over all cells in an epithelium are calculated. (6) This information is represented as a feature vector, which is an eight-dimensional vector that characterises each epithelium. Each of the four features considered in this work is abbreviated by the symbols shown in this figure. ( b ) Schematic representation of the comparisons of epithelia from different sources performed in this study. Images of representative epithelial samples (2-pixel wide cell contour) from Drosophila (different tones of green labels, fly) and chick (different tones of brown labels) are shown. The reference prepupal wing pouch epithelium is shown within a grey box. The text in grey denotes the relationship between epithelia from the different sources that were compared. Space : spatially separated epithelia from the same organism; time : temporally separated epithelia from different stages of development; type : different types of epithelia (that is, squamous and columnar); species : epithelia from different organisms (vertebrate (chick) and invertebrate ( Drosophila )) and mutation : mutant epithelia. Full size image For each type of epithelium, we collected a set of images from several different individuals and extracted the feature vectors in each case ( Supplementary Table S1 ). This allows us to compare epithelia, for example, from different developmental stages, tissues and species ( Fig. 1b ; Supplementary Figs S2 and S3 ), and the natural variation (that is, individual-to-individual variability) in epithelial organisation. To compare different epithelia, we used multivariate statistical methods to identify the contribution of the different features in the feature vector that best separate different epithelial types. We took advantage of an unsupervised and a supervised method, namely principal component analysis (PCA) and discriminant analysis (DA) [4] , [24] , [25] ( Box 1 ; Methods). Both these methods provide information about the relative contribution of the features that distinguish different epithelia, termed 'feature weights' ( Fig. 2a ; Supplementary Table S2 ). The statistical significance of the separation of the different epithelia was assessed using the multivariate analysis of variance (MANOVA) test (Methods). 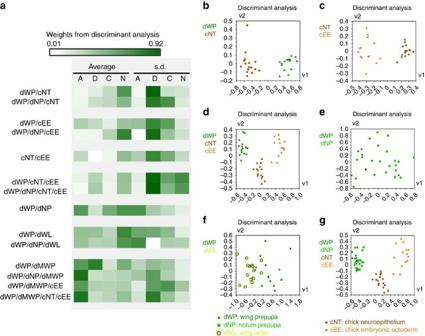Figure 2: DA of the different epithelia. (a) Colour-coded matrix representation of the weights of the features contributing to the observed projection in the DA of the different comparisons. A higher value (darker colour) represents a relatively higher contribution of the feature to the separation. (b–g) DA graphs of the comparisons of epithelia from different sources. (b) dWP-cNT. (c) cNT-cEE. (d) dWP-cNT-cEE. (e) dWP-dNP. (f) dWP-dWL. (g) dWP-dNP-cNT-cEE. v1 and v2 denote the first and second component of the projection. Figure 2: DA of the different epithelia. ( a ) Colour-coded matrix representation of the weights of the features contributing to the observed projection in the DA of the different comparisons. A higher value (darker colour) represents a relatively higher contribution of the feature to the separation. ( b – g ) DA graphs of the comparisons of epithelia from different sources. ( b ) dWP-cNT. ( c ) cNT-cEE. ( d ) dWP-cNT-cEE. ( e ) dWP-dNP. ( f ) dWP-dWL. ( g ) dWP-dNP-cNT-cEE. v1 and v2 denote the first and second component of the projection. Full size image Box 1: Qualitative definition of the geometric and network features and the statistical approaches used. Comparison of epithelia from different organisms To validate the approach, we first used the feature vector to compare visually distinct epithelia. For this, we took advantage of the neural tube (samples chick neuroepithelium (cNT1–cNT12) and chick embryonic ectoderm (cEE1–cEE14) from chicken embryos, and the Drosophila wing imaginal disc from the prepupal stage (dWP1–dWP16). DA and PCA revealed that the epithelia from the two different organisms could be clustered into two distinct groups ( Fig. 2b ; cNT and dWP; DA; P =9.17×10 −18 ; Supplementary Fig. S4 ; cEE and dWP; DA; P =2.41×10 −21 , Supplementary Fig. S5 ) demonstrating the efficacy of the method. The greater importance of the average degree of the neighbours (N) and the s.d. of the degree (D) in the dWP-cNT separation ( Fig. 2a,b ; Supplementary Table S1 ) suggest that these two network features capture a certain defining signature that is independent of the cell area (which is comparable for these epithelial types). Comparison of different epithelial types To verify whether we could discriminate between different types of epithelia from the same organism, we compared the cNT of the chick to the cEE. PCA and DA of the feature vectors of these two epithelia revealed that they form two distinct groups ( Fig. 2c ; DA; P =4.49×10 −16 ; Supplementary Fig. S6 ; PCA; P =4.27×10 −10 ). In this case, the cEE dataset was more spread out, reflecting the greater heterogeneity among these samples. However, each sample was clearly separated from cNT epithelia. In addition, the method separated the Drosophila wing pouch (dWP), the chick neuroepithelium (cNT) and embryonic ectoderm (cEE) epithelia into three groups ( Fig. 2d ), demonstrating that it is sensitive to different types of epithelial organisation. Multiple features contributed to the separation of these epithelia, suggesting that it was the combination of features that allowed the discrimination ( Fig. 2a ). This underscores the importance of global structure of the network. In particular, we found that the s.d. of the non-geometric (that is, network) features were more important in separating the different epithelial types, suggesting that, in this case, GNEO is able to capture patterns in epithelial organisation, which are not visually apparent and are independent of cell area. Comparison of epithelia from different developmental stages We next compared more closely related epithelia. DA on the feature vectors of the wild-type (WT) epithelia of the wing pouch (which develops into the adult wing blade; dWP1–dWP16) and the notum (which develops into the adult thorax; dNP1–dNP12) of the wing imaginal disc from the prepupal stage showed that these samples were only partially separable. This indicates a similarity in the overall organisation of both epithelia at this stage during development ( Fig. 2e ; DA; P =0.001), consistent with these regions comprising different areas of the same epithelial sheet. Moreover, a comparison of the prepupal wing pouch (dWP1–dWP16) with the third instar larva wing pouch (dWL1–dWL15) produced a discriminant graph with two groups, which also overlapped but were better separated ( Fig. 2f ; DA; P =3.45×10 −5 ) ( Supplementary Fig. S7 ). Together, these data suggest that the global organisation of the wing epithelia change gradually during development and across an epithelial sheet. The GNEO approach provides a way to assess the relatedness of different epithelia through approaches that calculate distances between data points using standard approaches such as hierarchical clustering. Consistent with our observation, a comparison of four epithelial types (DA and PCA of the Drosophila dWP and dNP, and the chick cEE and cNT) showed that dWP and dNP forms an overlapping cluster whereas the cEE and cNT form separate clusters ( Fig. 2g ). These observations confirm that the epithelial organisation of the prepupal notum and wing are similar whereas the neural tube and embryonic ectoderm are not. Comparison of epithelia from different tissues While the wing pouch and the notum are closely related, we tested if our approach can separate distantly related epithelia in Drosophila , by comparing the third instar larval wing disc epithelia (dWL) with the eye epithelia (dEL1–dEL5). Unlike the wing disc epithelium, the third instar eye disc contains a gradient of apical constriction induced by myosin II activation [26] , [27] , leading to apparently different cell shapes and sizes across the epithelial sheet. DA of the feature vectors clearly demonstrated that the eye and wing disc epithelia are significantly different and that most of the features, except the average clustering coefficient, contribute to this separation ( Supplementary Fig. S8 ; DA; P =1.11×10 −5 ). Natural variation in epithelial organisation The observation that the network features of the feature vectors were important in discriminating different types of epithelial tissues raised the possibility that local cell packing (resulting from cell shape and distribution) gives rise to the characteristic long-range patterns of an epithelium. In this view, the global organisation is a property of the epithelium that emerges from the collective behaviour of the cells. Consistent with this idea, the individual-to-individual variation (measured as coefficient of variation (c.v.), Table 1 and Methods) of mean values of the network features between the different individuals is several fold smaller than that of cell area ( Table 1 ). In addition, the individual-to-individual variation (c.v.) of the mean network features was much smaller than the c.v. of the cell-to-cell variability (that is, the s.d. of the features in the feature vector) across individuals. These observations suggest that there is a reproducible long-range epithelial structure, which is, to a large extent, independent of variations in cell size ( Table 1 ). Table 1 Coefficient of variation for the different features. Full size table Comparison of WT and genetically perturbed epithelia What regulates this reproducible long-range organisation of epithelia? Several factors have been implicated in controlling the behaviour of individual cells and consequently epithelial architecture [6] , [8] , [9] , [11] , [15] , [16] , [17] , [18] . However, how global epithelial structure is determined by, for example the effect of the cytoskeleton of the cells within the epithelium, is not understood. Therefore, we applied GNEO to quantify objectively the effect in the wing disc of removing myosin II heavy chain using RNAi [28] , [29] , a genetic manipulation that robustly and uniformly disrupts the cytoskeletal organisation and epithelial architecture (Methods). Both PCA and DA were clearly able to separate WT discs from those in which myosin II had been reduced ( Fig. 3a ; Supplementary Fig. S9a ). Interestingly, while all WT wings formed one distinct tight cluster, the mutant wings were more broadly spread over the graph ( Fig. 2a ; PCA; P =4.27×10 −10 ). This is consistent with a visual inspection of the data, which showed that reducing the levels of myosin II by RNAi knockdown disrupted epithelial organisation to different extents in different wing discs. In order to provide an objective score for the severity of the mutant phenotype, we calculated the Euclidean distance between each mutant wing and the centre of mass of the WT wings ( Supplementary Table S3 ). The c.v. of the distances was ∼ 26%, which most likely reflects the variability of the RNAi efficiency among the individuals. The individual mutant samples were between 15 and 35 times further from the centre of mass than the average of the distances of the dWP samples ( Supplementary Table S3 ). 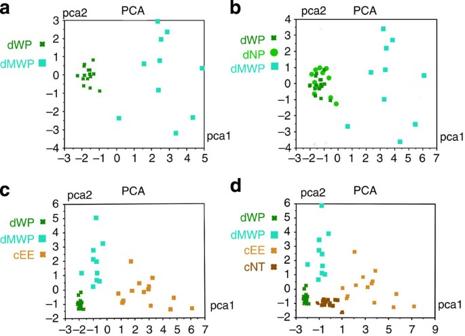Figure 3: PCA graphs of the WT and mutant epithelia. (a) dWP-dMWP. (b) dWP-dNP-dMWP. (c) dWP-dMWP-cEE. (d) dWP-dMWP-cEE-cNT. cEE, chick embryonic ectoderm; cNT, chick neural tube; dMWP, mutant wing prepupa; dWP, wing prepupa. Figure 3: PCA graphs of the WT and mutant epithelia. ( a ) dWP-dMWP. ( b ) dWP-dNP-dMWP. ( c ) dWP-dMWP-cEE. ( d ) dWP-dMWP-cEE-cNT. cEE, chick embryonic ectoderm; cNT, chick neural tube; dMWP, mutant wing prepupa; dWP, wing prepupa. Full size image We then investigated how the inclusion of other epithelia during the comparison affected our analysis of myosin II reduction. Addition of the prepupal notum (dNP) showed that both WT epithelia cluster together whereas the mutant wing pouch epithelia were still scattered ( Fig. 3b ; PCA; P =1.57×10 −13 and Supplementary Fig. S9b ; DA; P =1.89×10 −18 ). Thus, GNEO can objectively recognise that the Drosophila WT samples are similar to each other but distinct from the mutant ones. A PCA that includes the chick embryonic ectoderm and the neural tube, either together or alone, revealed that each group forms distinct clusters (PCA: Fig. 3c ; P =2.98×10 −31 ; Fig. 3d ; P =3.40×10 −22 and DA: Supplementary Fig. S9c ; P =2.03×10 −44 ; Supplementary Fig. S9d ; P =1.36×10 −34 ). This suggests that the Drosophila mutant epithelia are clearly distinct from the WT Drosophila and chick epithelia. DA indicated that the area, the degree, the degree of neighbours and the s.d. of the degree are the most important features ( Fig. 2a ) for obtaining this separation ( Supplementary Fig. S9a–d ). This is consistent with an effect of myosin II on regulating cell shape [26] , [27] , [30] , [31] , whose levels when altered affect cell area, the number of neighbours and the 'regularity' of the pattern of cell contacts. The increased variability of the network features when myosin II is knocked down demonstrating an important biological conclusion of this work: long-range constancy of epithelial packing is regulated by cytoskeletal organisation within individual cells. This is also reflected by the higher variation between discs from different individuals in the myosin II knockdown compared with WT discs ( Table 1 ). Together, these data suggest that the long-range organisation of an epithelium is determined, at least in part, by the cytoskeleton of the cells comprising the tissue affecting interactions across the field of cells. The network-based approach, GNEO, introduced here ( Fig. 1a ; Supplementary Fig. S9a ), captures epithelial organisation by accounting for patterns of cell contacts, which cannot be quantified either by visual inspection or by using geometric features that describe individual cells alone. In particular, GNEO can objectively quantify differences between epithelia from different tissues and organisms, even when the size and shape of the cells comprising these epithelia seem visually indistinguishable. First, we show that epithelia from different organs and species have distinct, reproducible and quantifiable differences in their structure. Second, a surprising result is that differences in cell area have a relatively minor role in distinguishing wing disc and neural tube epithelia—two epithelia that come from different species, which produce very different tissues. This indicates that there is unexpected consistency in both the average size and range of sizes of cells across epithelia from different species. Third, we provide evidence that the non-geometric features of the epithelia are most informative in distinguishing them. This shows that the topological organisation of the epithelium differs strongly between tissues and between species. Together with the finding that the structure of the same epithelia from different individuals is highly reproducible, our analysis indicates an unexpected level of genetic control over the long-range organisation of epithelia. To the best of our knowledge, this has not been previously reported. Lewis's and Aboav-Weaire's laws [23] define relationships between area, degree and neighbour degree, and place the emphasis on the universal connection between these features. By contrast, our work examines how measurements of these features across a population of cells can be used to build a quantitative and objective description of an epithelium. The experiment in which we disrupt myosin II provides an indication of the mechanism by which population level features of an epithelium emerge from the collective behaviour of individual cells. Moreover, we provide evidence that GNEO can operate as a reliable classifier to differentiate mutant and WT epithelia, and to quantify precisely the severity of mutant phenotypes. While there are other ways of constructing networks from images of epithelia, this representation of cell-to-cell contacts offers a simple and readily applicable method to analyse epithelia objectively. Representing epithelia as feature vectors opens up the possibility of applying artificial intelligence (for example, pattern recognition) algorithms to classify them in an objective manner and can be extended to include more sophisticated network features. As the method is automatable, adaptations of this approach can be used in high-throughput experiments aimed at identifying pathways and quantifying the effects of mutations in functional genomics screens. Of particular value, GNEO allows characterisation of subtle phenotypes undetectable by visual inspection. This approach can also be adapted to other biological samples such as nerve–cell connections, muscle cells attachments and tumours. Genetic strains and confocal imaging of the epithelia Flies were grown by employing standard culture techniques. The following lines were used: Arm-GFP (WT), C765-Gal4 ( http://flybase.bio.indiana.edu ) and U-zip-RNAi (Vienna Drosophila RNAi Center collection). Imaginal discs from the prepupa and third instar larvae were dissected in PBS and fixed with 4% paraformaldehyde in PBS for 35 min. The samples were washed six times for 10 min with PBT (PBS, 0.3% triton) and 3 times for 5 min with PBS. Imaginal discs were mounted using Fluoromount-G (Southern Biotech). Images were taken with a BioRad Radiance 2,100 laser scanning confocal microscope (BioRad). All the images were captured using X63 immersions objective with three times zoom and exported as a 1,024×1,024 pixel TIFF file. The area of 1 pixel is 3.78×10 −3 μm 2 . The regions of the imaginal discs that seem in the images were selected with the following criteria: For the prepupal and larval wing disc, images from dorsal compartments (leaving out the D/V boundary region) of the wing pouch region were obtained. The notum images were taken from the anterior part of the disc ( Supplementary Fig. S2 ). For the eye disc, the images were taken locating the morphogenetic furrow at the side with an additional margin of three to five rows of cells (to include the first and second rows of clusters of photoreceptors). For the chick images, Hamburger and Hamilton (HH) [32] stage 10 and 17 chick embryos ( Supplementary Fig. S3 ) were fixed for 1 h in 4% paraformaldehyde. HH stage 17 embryos were subsequently transferred to methanol, then rehydrated. Immunostaining was performed with a ZO1 antibody (Zymed labs), and embryos were flat mounted. Images of neural tube epithelium, at intermediate dorsoventral positions, were obtained at the level of somite 5 of HH stage 17 embryos. Embryonic ectoderm was imaged adjacent to the most recently formed somite of HH stage 10 embryos. Imaging conditions were as for imaginal discs, image orientation: anterior, left; dorsal, up. Image processing and generation of the epithelial network The acquired images were converted into their respective 2-pixel BMP files ( Supplementary Data 1 , 2 , 3 , 4 , 5 , 6 , 7 ). First, the confocal images were imported using Adobe Photoshop CS2. Colours were inverted to obtain a dark signal over a light background. Epithelial cells were identified from the processed images by using a semiautomated framework. The images first had their illumination corrected through polynomial fitting followed by thresholding, and were then manually checked and edited to remove artefactual connections between cells. The cells and their boundaries were defined using a foreground tracking program [4] . Adjacent cells were identified by transforming their images into an epithelial network where the centroid of each cell is represented by a node and the neighbourhood relations are mapped into weighted edges ( Supplementary Fig. S1 ). The methodology involves the following steps: (a) all cells have their borders detected [4] , (b) for each pixel p of the border of each cell i , all border pixels belonging to other cells and falling within the circle of radius r centred at p are identified and counted (we use r =6) and (c) the node corresponding to this cell is connected to other cells by edges whose weights, w , correspond to the total number of neighbouring pixels found during step (b). We established empirically that if the weight is greater than 40% of the minimum equivalent radius of the areas of each adjacent pair of cells, those cells can be considered to be neighbours. The equivalent radius of a cell with area A is defined as corresponding to We selected an area within every image in order to have all the networks presented with similar boundary conditions. The squares were drawn to obtain the maximum possible surface without including the centroids of the cells in the border of the images. The features of the cells falling within this area were calculated. The cells outside were only used in order to provide neighbours to the cells analysed in the network. Calculation of geometric and network features The area was measured by counting the number of pixels inside each cell [4] . Each epithelial image was represented as a network where each node corresponds to one of the cells, and the links between nodes reflect the spatial adjacency between the epithelial cells ( Fig. 1a ). Several measurements can be estimated from these networks [24] , in order to provide useful characterisation and respective biological interpretations. Let the graph be represented in terms of its adjacency matrix K , such that the presence of a connection between nodes i and j , with 1≤ i , j ≤ N , implies K ( i , j )= K ( j , i )=1, with K ( i , j )= K ( j , i )=0 being enforced otherwise. In this work, we employed the following topological characteristics: degree of a node i , which corresponds to the number of edges attached to it, that is, Clustering coefficient of a node i , which is obtained by dividing the number of edges between the neighbours of i , represented as n ( i ), by the maximum possible number of connections between those nodes. This measurement can be calculated as Therefore, the clustering coefficient varies from 0 (no interconnections between the neighbours of i ) to 1 (the neighbours are fully interconnected). Average degree of the neighbours of a node, calculated as the average of the number of edges that are attached to the neighbours of node i . This measurement can be calculated as For every feature, both the average and s.d. values across all cells in an epithelium were estimated and were used to characterise epithelial organisation. Cell elongation was initially considered as an independent parameter but was found not to contribute further to the classification and separation. We believe that this is because variations in the elongation tend to affect the degree, clustering coefficient and average degree of neighbours, therefore becoming correlated with those measurements. All software were written in house ( Supplementary Software 1 , 2 , 3 , 4 , 5 ). Feature vector and multivariate statistical analysis The geometric and network analyses of epithelial images yield a large number of features or measurements ( Supplementary Table S1 ). More precisely, a total of eight features, corresponding to the mean and s.d. of the area of cells, as well as the degree, clustering coefficient and average degree of a node are obtained. Thus, for every image of an epithelium, a feature vector of eight dimensions was obtained. We apply an unsupervised and supervised multivariate statistical method, namely PCA and DA [4] , [24] , [25] ( Supplementary Methods ). Standardisation [4] of the measurements is performed in order to eliminate the effect of the magnitude of the measurements on the respective separation between categories. More specifically, the average and s.d. for every feature across all individuals in each of the epithelial type was calculated. For every feature in a feature vector representing an individual epithelium, the calculated average value was subtracted and divided by the s.d. Thus, the components of the eigenvectors associated to the largest eigenvalues provide a quantification of the degree of contribution of each original measurement in maximising the dispersion of the projection (in the case of PCA) and optimising the separation between the categories (in the case of DA). As both these methods output a weighted linear combination of all the features in the feature vector to obtain the final projection (the new axes), the loading values associated to each feature provide a direct measure of the contribution of that particular feature towards the projection onto the smaller-dimensional space. For our analysis, the maximum between the magnitudes of the values of the components of each feature (that is, measurement) of the first two eigenvector (that is, the loadings associated with the first two component axes) was defined as the weight of that respective measurement. Estimation of statistical significance The MANOVA test, which is a reference statistical test for probing the hypotheses that two or more populations, characterised in terms of two or more dependent variables, are or not distinct, was used to assess the statistical significance of the obtained separation. The tested (null) hypothesis H0 is that the two samples come from the same population, with H1 indicating different populations. The P -values are calculated in the standard way [33] , [34] , after PCA or DA. Both PCA and DA provide new random variables that are linear combinations of the previous ones. In the case of PCA, the new variables are completely uncorrelated. In the case of DA, the method does take into account the known categories of the cells and therefore enhances the separation between the categories. In this case, our interest was focused on the contribution of the measurements on the separation, not on the separation itself. The P -values in this case reflect the effect of the informed cell categories and should be treated as such. The assumptions required for MANOVA were verified even though after application of PCA and DA, as the respective clusters remained largely normal and with similar variances. How to cite this article: Escudero, L.M. et al . Epithelial organisation revealed by a network of cellular contacts. Nat. Commun. 2:526 doi: 10.1038/ncomms1536 (2011).